A kinase inhibitor screen identifies small-molecule enhancers of reprogramming and iPS cell generation Somatic cells can be reprogrammed to form embryonic stem cell-like induced pluripotent stem cells (iPSCs), but the process suffers from low efficiency and the underlying molecular mechanisms that control reprogramming remain poorly understood. Here we perform an inhibitor screen to identify kinases that enhance, or present a barrier to, reprogramming. In particular, inhibitors of p38, inositol trisphosphate 3-kinase, and Aurora A kinase potently enhance iPSC generation, and iPSCs derived from inhibitor-treated somatic cells are capable of reaching a fully reprogrammed state. Knockdown of target kinases by short interfering RNAs confirms that they function as barrier genes. We show that Aurora A kinase, which functions in centrosome activity and spindle assembly, is highly induced during reprogramming and inhibits Akt-mediated inactivation of GSK3β, resulting in compromised reprogramming efficiency. Together, our results not only identify new compounds that enhance iPSC generation but also shed new light on the function of Aurora A kinase in the reprogramming process. Since the original discovery that ectopic expression of four transcription factors (Oct4, Klf4, Sox2 and c-Myc) can create cells closely resembling embryonic stem cells (ESCs), various types of mouse and human somatic cells have been reprogrammed to establish induced pluripotent stem cells (iPSCs) [1] , [2] , [3] , [4] , [5] , which have the capacity to differentiate into different cell lineages [3] , [4] , [5] . The differentiated cells are reportedly functional in vitro and in vivo and have been shown to correct various diseases in mouse models [6] . Moreover, iPSCs have been generated from tissues of patients with different diseases and could thus be a valuable resource to study disease pathology or for drug screening in vitro [7] , [8] , [9] , [10] . Despite the promise of in vitro reprogramming, the process suffers from extremely low efficiency [1] , [2] , [11] , [12] . Thus, there is a need to better understand the molecular events underlying reprogramming and to develop more efficient methods to generate iPSCs. A number of elegant approaches have been taken to identify the critical pathways that regulate reprogramming. For example, cells at different stages of reprogramming, including the starting somatic cells, the derived iPSCs and various intermediate cell populations, have been subjected to mRNA profiling. These studies have indicated that cells can become 'trapped' in a partially reprogrammed state and that treatment with DNA methyltransferase inhibitors enables them to become fully reprogrammed [13] . The notion that DNA binding and gene activation are altered in partially reprogrammed iPSCs is supported by genome-wide analysis of promoter binding by specific transcription factors [14] . Moreover, several groups have shown that the p53 pathway, which is activated following overexpression of the oncogenic reprogramming factors, acts as a major reprogramming barrier [15] , [16] , [17] , [18] . Recent studies showed that transforming growth factor (TGF)-β signalling also inhibits reprogramming [19] , [20] and perturbs the mesenchymal-to-epithelial transition [21] , [22] , a process that enhances reprogramming and is regulated by microRNAs [23] . Nonetheless, in relative terms little is known about how terminally differentiated cells are reprogrammed to an ESC-like state by the four transcription factors. In recent years, there has been a concerted effort to identify agents that can enhance iPSC derivation. In addition to small molecules that can reportedly replace one or more of the four reprogramming factors [20] , [24] , [25] , [26] , other compounds have been shown to enhance the efficiency of four-factor (4F) reprogramming; namely, TGF-β receptor inhibitors, 5-aza-cytidine, vitamin C and valproic acid [13] , [19] , [27] , [28] . Although some investigators report that valproic acid treatment dramatically enhances iPSC generation, more recent reports have reexamined the effects and found them to be modest [29] , [30] , [31] . Therefore, only a limited number of compounds are currently known to enhance iPSC generation. Kinases promote phosphorylation of targets by transferring phosphate groups from high-energy donors, usually ATP. Kinases are of great importance in maintaining cellular homeostasis, and they regulate many key processes including the cell cycle and metabolic switching [32] , [33] . However, few kinases have been shown to function in the reprogramming process [34] . Given their critical function in numerous signalling pathways, we hypothesized that kinases may be involved in the reprogramming process and that their activity might be manipulated to enhance iPSC generation. Here we report the results of an inhibitor screen designed to identify both barrier and essential kinases that function in reprogramming. We found that the essential kinases were enriched in cell cycle and proliferation regulators, whereas three kinases, p38, inositol trisphosphate 3-kinase (IP3K) and Aurora A kinase, were identified as new barrier genes. Accordingly, iPSC generation was significantly enhanced by inhibiting the function of these barrier kinases with small molecules. iPSCs derived from inhibitor-treated mouse embryonic fibroblasts (MEFs) reached a fully reprogrammed state and differentiated into different lineages in vitro and in vivo . The specificity of the inhibitors was confirmed using independently validated inhibitors and RNA interference-mediated knockdown of the kinases. Moreover, we found that Aurora A kinase functions to inhibit Akt-mediated GSK3β phosphorylation, which maintains GSK3β in an active state. GSK3β inhibition has been reported to enhance somatic cell reprogramming efficiency [35] . To our knowledge, this is the first report of a function for Aurora A kinase beyond its characterized role in centrosome formation and spindle assembly. Overall, our data provide new insights into the mechanisms underlying reprogramming and identify inhibitors that could significantly enhance iPSC generation. Identification of small molecules that alter iPSC generation To define signalling mechanisms underlying reprogramming, we undertook a double-blind screen of 244 well-characterized cell-permeable protein kinase inhibitors to identify kinases that enhance or inhibit the process. As the starting material, we used MEFs from a transgenic line in which green fluorescent protein (GFP) expression is driven by the endogenous Oct4 promoter. Endogenous Oct4 expression is switched on in fully reprogrammed cells; thus, the reprogramming efficiency can be quantified by counting GFP+ iPSC colonies. To minimize well-to-well variation, MEFs were first retrovirally transduced with the 4F in bulk ( Fig. 1a ) and then reseeded at 3,000 cells per well in gelatin-coated 96-well plates before treatment with inhibitors. Starting on day 3 post-transduction, inhibitors were added at a final concentration of 2 μM. Medium was replaced every other day with fresh mouse embryonic stem cell (mES/mESC) medium containing 2 μM of the appropriate inhibitor. On day 13 post-transduction, cells were fixed in 4% paraformaldehyde and GFP+ colonies were quantified by microscopy. 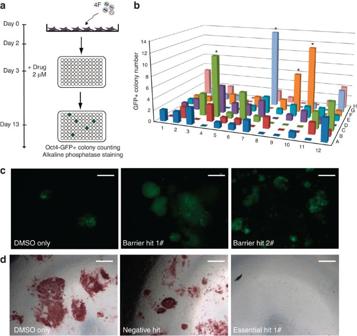Figure 1: A kinase inhibitor library screen identifies essential and barrier kinases. (a) Design of the screen. MEFs were transduced with the four mouse-reprogramming factors (4F) for 2 days and reseeded into 96-well plates. Drugs were added at a final concentration of 2 μM on day 3. The medium was changed every other day until day 13, when cells were collected for colony counting and AP staining. (b) Representative 96-well plate showing quantification of Oct4-GFP+ colonies. GFP+ colonies were counted directly under a fluorescence microscope. *Indicates an identified hit. Columns 1 and 12 contain control DMSO-treated cells. Potential candidates were determined by GFP+ colony number, morphology and AP staining. (c) Representative barrier kinase hits. Oct4-GFP+ colony numbers were dramatically increased following treatment with some of the inhibitors. GFP+ colonies were quantified and images were taken on day 14 post-4F transduction. Scale bar, 200 μm. (d) Representative hits of essential kinases. Essential hits were identified by loss of AP staining in the absence of cell death. Scale bar, 200 μm. Figure 1: A kinase inhibitor library screen identifies essential and barrier kinases. ( a ) Design of the screen. MEFs were transduced with the four mouse-reprogramming factors (4F) for 2 days and reseeded into 96-well plates. Drugs were added at a final concentration of 2 μM on day 3. The medium was changed every other day until day 13, when cells were collected for colony counting and AP staining. ( b ) Representative 96-well plate showing quantification of Oct4-GFP+ colonies. GFP+ colonies were counted directly under a fluorescence microscope. *Indicates an identified hit. Columns 1 and 12 contain control DMSO-treated cells. Potential candidates were determined by GFP+ colony number, morphology and AP staining. ( c ) Representative barrier kinase hits. Oct4-GFP+ colony numbers were dramatically increased following treatment with some of the inhibitors. GFP+ colonies were quantified and images were taken on day 14 post-4F transduction. Scale bar, 200 μm. ( d ) Representative hits of essential kinases. Essential hits were identified by loss of AP staining in the absence of cell death. Scale bar, 200 μm. Full size image Two columns of wells from each plate (columns 1 and 12) were treated with dimethylsulphoxide (DMSO, vehicle) only and served as controls. On average, the control wells contained two to three GFP+ colonies per well, which was around 0.07% reprogramming efficiency and was comparable to the efficiency reported by others [1] , [2] , [11] , [12] . To identify inhibitors that significantly enhanced reprogramming efficiency, we set a minimum threshold filter of a 2.5-fold increase in GFP+ colony number. Using these criteria, we identified 11 inhibitors as 'barrier hits' or potential activators of reprogramming ( Fig. 1b,c ; Table 1 ). Because kinases may also be required for iPSC generation, we performed alkaline phosphatase (AP) staining for iPSCs to identify inhibitors as potential 'essential hits'. As genes encoding targets of essential hits could function at various reprogramming stages and most cells did not attain a fully reprogrammed state, we used a stringent criterion to identify essential hits: wells were scored positive only if they were devoid of AP+ cells and had no obvious decrease in cell number ( Fig. 1d ). Nine kinase inhibitors were identified as essential hits according to these standards ( Supplementary Table S1 ), and further analysis revealed that four of them were direct inhibitors of cell cycle-dependent kinases (Cdks), indicating that cell cycle control is critical for reprogramming. We tested four of the remaining essential hits ( Supplementary Fig. S1a ) and found that three hits inhibited MEF proliferation to various extents with or without 4F transduction ( Supplementary Fig. S1b,c ) and decreased reprogramming efficiency in direct proportion to their effects on proliferation ( Supplementary Fig. S1d ). Overall, these findings suggest that the reduction in reprogramming efficiency following inhibition of essential kinases correlates with the effects on MEF proliferation. Table 1 Small molecule enhancers of iPSC generation. Full size table Select inhibitors significantly enhance reprogramming To confirm that the 11 barrier hits ( Table 1 ) identified in the primary screen are able to enhance iPSC generation, we undertook a secondary screen using larger wells and two drug concentrations (1 and 2 μM). These analyses confirmed that 4 of the 11 barrier candidates ( Fig. 2a ), B4, B6, B8 and B10, consistently and significantly enhanced reprogramming and had greater effects at the lower concentration of 1 μM than at 2 μM ( Fig. 2b ). In addition, B8 and B10 enhanced iPSC generation even under non-permissive conditions, in which 4F expression was too low to reprogram vehicle-treated MEFs ( Supplementary Fig. S2a ). Two other groups recently identified the inhibitor B4 as being able to enhance reprogramming and/or replace Sox2 in the 4F cocktail [19] , [20] . Additional dose–response analyses confirmed that B6, B8 and B10 act as potent enhancers at concentrations as low as 0.5 μM ( Supplementary Fig. S2b ). Moreover, these inhibitors did not significantly promote proliferation of either uninfected or 4F-transduced MEFs ( Supplementary Fig. S2c,d ). When combined at 1 μM each, B6, B8 and B10 had a synergistic rather than an additive effect on reprogramming efficiency ( Supplementary Fig. S2e ). Because p53 has previously been identified as a major barrier to reprogramming [15] , [16] , [17] , [18] , [36] , we asked whether B6, B8 or B10 enhanced reprogramming following short hairpin RNA-mediated downregulation of p53. As expected, p53 knockdown in 4F-transduced MEFs greatly enhanced iPSC generation, but this enhancement was unaffected by treatment with B6, B8 or B10 ( Supplementary Fig. S2f,g ). 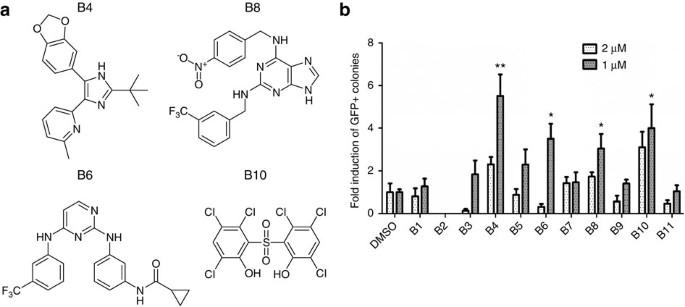Figure 2: Inhibitors of several target kinases greatly enhance iPSC generation. (a) Chemical structures of B4, B6, B8 and B10. (b) Compounds B4, B6, B8 and B10 significantly enhanced reprogramming. Drugs were added at 1 or 2 μM on day 3 post-4F transduction and Oct4-GFP+ colonies were quantified 10 days later. Notably, B6 showed enhancement only at the lower dose (1 μM). Data are mean±s.d. and are representative of three independent experiments. *P<0.05; **P<0.01 (Studentt-test). Figure 2: Inhibitors of several target kinases greatly enhance iPSC generation. ( a ) Chemical structures of B4, B6, B8 and B10. ( b ) Compounds B4, B6, B8 and B10 significantly enhanced reprogramming. Drugs were added at 1 or 2 μM on day 3 post-4F transduction and Oct4-GFP+ colonies were quantified 10 days later. Notably, B6 showed enhancement only at the lower dose (1 μM). Data are mean±s.d. and are representative of three independent experiments. * P <0.05; ** P <0.01 (Student t -test). Full size image It is possible that B6, B8 and B10 could target multiple kinases; therefore, we validated the specificities of these compounds by RNA interference experiments. To do this, MEFs and mESCs were transfected with short interfering RNAs (siRNAs) specific for potential targets of each inhibitor and the knockdown efficiencies were evaluated by reverse transcription–quantitative PCR (RT–qPCR). Indeed, all siRNAs tested efficiently knocked down their target genes in MEFs ( Fig. 3a,b ) and in mESCs ( Fig. 3b ). We next transfected MEFs with these siRNAs and 3 h later transduced the cells with 4F. GFP+ colonies were counted ~12 days post 4F transduction. Of note, we found that Mapk11 (p38β; a target of inhibitor B10), ItpkA (a target of inhibitor B8), Stk6 (Aurora A kinase) and Syk (targets of inhibitor B6) act as barrier genes: knockdown of any one of these genes during reprogramming resulted in a significant increase in iPSC generation ( Fig. 3c,d ). Interestingly, knockdown of some B6 targets, such as Bmx, Igf1r and Lck, actually compromised reprogramming, which may at least partially explain how B6 inhibits or enhances reprogramming at different concentrations. Together, these data confirm that inhibitors B4, B6, B8 and B10 ( Fig. 2a ) are potent enhancers of iPSC generation and that they act in a target-specific manner. 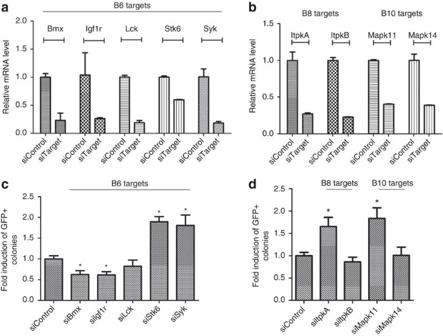Figure 3: Inhibitor-targeted kinases are confirmed as barrier genes. (a,b) Potential targets of B6, B8 and B10 inhibitors were knocked down by siRNAs in MEFs or mESCs (ItpkA only). Cells were transfected with 50 nM siRNAs and total RNA was collected 2 days later for RT–qPCR analysis. Error bar represents variation of duplicate wells. (c) Potential targets of B6 were knocked down by siRNAs and reprogramming efficiency was quantified by counting Oct4-GFP+ colonies. Data are mean±s.d. from three independent experiments and were normalized to short interfering (si) Control-transfected samples. *P<0.01 (Student'st-test). (d) Knockdown of B8 and B10 targets enhances reprogramming. Data are mean±s.d. from three independent experiments and were normalized to siControl-transfected cells. Figure 3: Inhibitor-targeted kinases are confirmed as barrier genes. ( a , b ) Potential targets of B6, B8 and B10 inhibitors were knocked down by siRNAs in MEFs or mESCs (ItpkA only). Cells were transfected with 50 nM siRNAs and total RNA was collected 2 days later for RT–qPCR analysis. Error bar represents variation of duplicate wells. ( c ) Potential targets of B6 were knocked down by siRNAs and reprogramming efficiency was quantified by counting Oct4-GFP+ colonies. Data are mean±s.d. from three independent experiments and were normalized to short interfering (si) Control-transfected samples. * P <0.01 (Student's t -test). ( d ) Knockdown of B8 and B10 targets enhances reprogramming. Data are mean±s.d. from three independent experiments and were normalized to siControl-transfected cells. Full size image Inhibitor-treated iPSCs reach a fully reprogrammed state Although B6, B8 and B10 promote reprogramming, it is possible that cells treated with these inhibitors turn on endogenous Oct4 expression but do not reach a fully reprogrammed state. To exclude this possibility, iPSCs derived from cells treated with each inhibitor were analysed for mESC marker expression and functional pluripotency. All GFP+ clones were also AP+ ( Fig. 4a ). Immunostaining for other mESC self-renewal markers confirmed that the inhibitor-derived iPSCs expressed Nanog and the mESC-specific surface protein SSEA1 ( Fig. 4b ). Moreover, genome-wide mRNA expression profiling verified that these cells showed a gene expression pattern highly similar to that of mESCs and significantly different from that of the starting MEFs ( Fig. 4c ). To determine whether inhibitor-treated cells acquire the full capacity to differentiate into different lineages, we used in vitro embryoid body (EB) formation assay to assess pluripotency. The inhibitor-treated iPSC clones readily differentiated into the three major lineages, including beating cardiomyocytes ( Supplementary Movie 1–3 ), and EBs stained positively for AFP (endoderm), tubulin III (ectoderm) and cardiac actin (mesoderm; Supplementary Fig. S3 ). To test pluripotency more stringently, we injected the inhibitor-treated iPSCs into athymic nude mice and found that all tested clones generated heterogeneous teratomas within 3–4 weeks ( Fig. 4d ). Moreover, iPSCs injected into the cavity of recipient blastocysts had successfully integrated with cells of the inner cell mass by the following day ( Supplementary Fig. S4a,b ) and contributed to living chimeric mice ( Fig. 4e ). These cells also contributed to the germ line of E13.5 embryos, suggesting that they were germ line competent ( Supplementary Fig. S4c ). Collectively, these data strongly suggest that iPSCs derived from inhibitor-treated MEFs are fully reprogrammed and are able to differentiate into all lineages in vitro and in vivo . 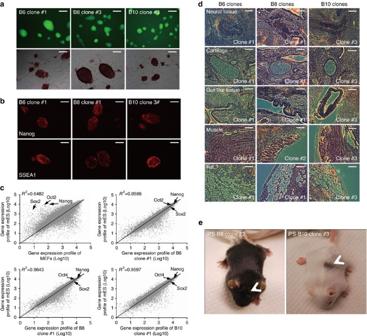Figure 4: Inhibitor-treated iPSCs reach a fully reprogrammed state. (a) iPSC clones from inhibitor-treated samples were picked and expanded. Cells show endogenous Oct4 expression (upper panels) and AP positivity (lower panels). Scale bar, 100 nm. (b) Inhibitor-treated iPSCs are Nanog+ and SSEA1+. iPSCs were seeded on irradiated MEF plates and cultured for 3 days, fixed in 4% paraformaldehyde and stained for Nanog and SSEA1 expression (seeSupplementary Methods). Scale bar, 100 μm. (c) Genome-wide mRNA expression profiles of derived iPSCs. B6-, B8- and B10-treated iPSC clones show expression profiles resembling that of control mESCs (CCE;R2>0.95). (d) iPSC clones derived from inhibitor-treated cells were injected into athymic nude mice and the tumours were collected after ~3 weeks. Scale bar, 200 μm. (e) Inhibitor-treated iPSCs can contribute to chimeric mice. Arrows indicate the altered coat colour, representing the contribution of injected iPSCs to the chimeric mice. Figure 4: Inhibitor-treated iPSCs reach a fully reprogrammed state. ( a ) iPSC clones from inhibitor-treated samples were picked and expanded. Cells show endogenous Oct4 expression (upper panels) and AP positivity (lower panels). Scale bar, 100 nm. ( b ) Inhibitor-treated iPSCs are Nanog+ and SSEA1+. iPSCs were seeded on irradiated MEF plates and cultured for 3 days, fixed in 4% paraformaldehyde and stained for Nanog and SSEA1 expression (see Supplementary Methods ). Scale bar, 100 μm. ( c ) Genome-wide mRNA expression profiles of derived iPSCs. B6-, B8- and B10-treated iPSC clones show expression profiles resembling that of control mESCs (CCE; R 2 >0.95). ( d ) iPSC clones derived from inhibitor-treated cells were injected into athymic nude mice and the tumours were collected after ~3 weeks. Scale bar, 200 μm. ( e ) Inhibitor-treated iPSCs can contribute to chimeric mice. Arrows indicate the altered coat colour, representing the contribution of injected iPSCs to the chimeric mice. Full size image Aurora A inhibition enhances Akt-mediated GSK3β inactivation To identify the mechanism by which kinase inhibitors might enhance reprogramming, the B6 target Aurora A kinase (AurkA) was chosen for further analysis because it has well-known functions in cell cycle progression, spindle formation and tumour development [33] . We first determined whether B6 treatment affected levels of AurkA protein and found B6 treatment of both wild-type and 4F-infected MEFs increased AurkA protein levels relative to untreated cells ( Fig. 5a ). In addition, 4F infection alone significantly increased AurkA protein levels compared with uninfected cells. Further experiments suggested that this increase could be due to enhanced transcription because AurkA mRNA was induced by approximately three- to fourfold in both untreated and DMSO-treated 4F-infected cells relative to the equivalently treated uninfected MEFs ( Fig. 5b ), and mRNA levels were not significantly altered by B6 treatment ( Fig. 5b ). These results agree with previous expression profiling studies of MEFs and iPSCs [14] , which showed that AurkA mRNA is highly expressed in mESCs or iPSCs compared with MEFs. During reprogramming with 4F, we also noted that levels of phosphorylated GSK3β decreased, indicating that GSK3β is activated. Interestingly, recent studies showed that inhibition of GSK3β by small molecules enhances iPSC generation from neural stem cells [35] . Therefore, we asked whether AurkA inhibition by B6 affected GSK3β phosphorylation. Indeed, we detected a significant increase in phospho-GSK3β in B6-treated cells ( Fig. 5c ), whereas total GSK3β protein level was unchanged. To confirm the specificity of the B6 effect on GSK3β phosphorylation, we assessed reprogramming in the presence of a different AurkA inhibitor, MLN8237, which has been demonstrated to have a potent inhibitory effect on AurkA in myeloma cell lines [37] . MLN8237 treatment also increased AurkA protein levels ( Fig. 5d ) and AurkA inhibition promoted a dose-dependent increase in the appearance of phospho-GSK3β but had no effect on total GSK3β levels ( Fig. 5d ). Collectively, these results indicate that AurkA inhibition promotes phosphorylation and subsequent inactivation of GSK3β, an effect that likely enhances reprogramming. 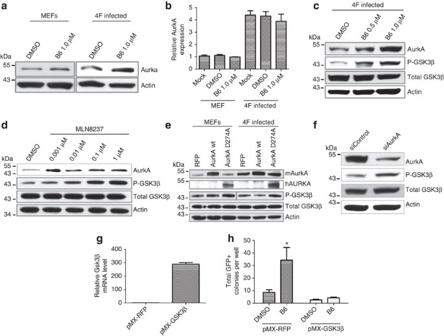Figure 5: Inhibition of Aurora A kinase by B6 promotes inactivation of GSK3β. (a) Both mock-infected and 4F-infected (day 3) MEFs were treated with 1 μM B6 for 2 days and then collected for western blotting of AurkA. Actin served as a loading control. (b) MEFs were infected with 4F for 3 days and mock-treated or treated with DMSO or 1 μM B6 for 2 days before isolation of total RNA and RT–qPCR analysis. B6 treatment did not alter induction of AurkA by 4F. Error bar represents variation between two experiments with triplicate wells. (c) 4F-infected MEFs were treated with the indicated doses of B6 inhibitor starting on day 3 post-infection and 2 days later were collected for western blotting analysis. (d) Inhibition of AurkA by MLN8237 also increases AurkA protein level and dose-dependently promotes GSK3β phosphorylation. The experiment was performed the same as forc. Actin served as the loading control. (e) Expression of a dominant-negative form of AurkA promotes GSK3β (Ser9) phosphorylation. MEFs were infected with 4F plus expression vectors for red fluorescent protein (RFP), wild-type (wt) murine AurkA or the D274A kinase-dead mutant of human AurkA. Expression of wt AurkA inhibited GSK3β phosphorylation on Ser9, whereas overexpression of the mutant AurkA D274A enhanced GSK3β phosphorylation. Exposure time was almost doubled for 4F-infected samples. (f) MEFs were transfected with 50 nM AurkA and control siRNAs for 2 days. Cells were then collected for western blotting of AurkA, total and phosphorylated GSK3β (Ser9), and actin as a loading control. (g) MEFs were infected with pMX-RFP (control) or pMX-GSK3β virus for 4 days and then collected for RT–qPCR analysis. Error bar represents variation of duplicate wells. (h) Overexpression of GSK3β blocked the effect of B6 on reprogramming. pMX-Gsk3β was transduced into MEFs together with 4F viruses. B6 (1 μM) was added at day 3 post-transduction and GFP+ colonies were quantified on day 12 post-transduction. Data are mean±s.d. of three independent wells. *P<0.05 (Student'st-test). Figure 5: Inhibition of Aurora A kinase by B6 promotes inactivation of GSK3β. ( a ) Both mock-infected and 4F-infected (day 3) MEFs were treated with 1 μM B6 for 2 days and then collected for western blotting of AurkA. Actin served as a loading control. ( b ) MEFs were infected with 4F for 3 days and mock-treated or treated with DMSO or 1 μM B6 for 2 days before isolation of total RNA and RT–qPCR analysis. B6 treatment did not alter induction of AurkA by 4F. Error bar represents variation between two experiments with triplicate wells. ( c ) 4F-infected MEFs were treated with the indicated doses of B6 inhibitor starting on day 3 post-infection and 2 days later were collected for western blotting analysis. ( d ) Inhibition of AurkA by MLN8237 also increases AurkA protein level and dose-dependently promotes GSK3β phosphorylation. The experiment was performed the same as for c . Actin served as the loading control. ( e ) Expression of a dominant-negative form of AurkA promotes GSK3β (Ser9) phosphorylation. MEFs were infected with 4F plus expression vectors for red fluorescent protein (RFP), wild-type (wt) murine AurkA or the D274A kinase-dead mutant of human AurkA. Expression of wt AurkA inhibited GSK3β phosphorylation on Ser9, whereas overexpression of the mutant AurkA D274A enhanced GSK3β phosphorylation. Exposure time was almost doubled for 4F-infected samples. ( f ) MEFs were transfected with 50 nM AurkA and control siRNAs for 2 days. Cells were then collected for western blotting of AurkA, total and phosphorylated GSK3β (Ser9), and actin as a loading control. ( g ) MEFs were infected with pMX-RFP (control) or pMX-GSK3β virus for 4 days and then collected for RT–qPCR analysis. Error bar represents variation of duplicate wells. ( h ) Overexpression of GSK3β blocked the effect of B6 on reprogramming. pMX-Gsk3β was transduced into MEFs together with 4F viruses. B6 (1 μM) was added at day 3 post-transduction and GFP+ colonies were quantified on day 12 post-transduction. Data are mean±s.d. of three independent wells. * P <0.05 (Student's t -test). Full size image AurkA reportedly has a kinase-independent function [38] . We therefore asked whether the kinase activity of AurkA is required for its inactivation of GSK3β. To address this, we overexpressed AurkA in 4F-infected MEFs using two retroviral constructs: one encoding wild-type mouse AurkA and the second encoding a kinase-dead mutant (D274A) of human AurkA [38] ( Fig. 5e , Supplementary Fig. S5 ; note that AurkA is highly conserved between humans and mouse). If the inactivation of GSK3β induced by B6 treatment is independent of AurkA enzymatic activity, we expected that overexpression of either construct should decrease GSK3β phosphorylation. However, if AurkA kinase activity was necessary for this effect, overexpression of the kinase-dead mutant should have a dominant-negative effect, similar to small molecule-mediated inhibition of AurkA activity. Indeed, we detected a significant increase in phospho-GSK3β levels in both 4F-infected and untreated MEFs expressing the kinase-dead mutant ( Fig. 5e ). In contrast, overexpression of wild-type AurkA decreased phospho-GSK3β without altering total protein levels ( Fig. 5e ). As expected, AurkA knockdown by siRNAs in MEFs also enhanced GSK3β phosphorylation ( Fig. 5f ). Finally, overexpression of GSK3β in MEFs largely abolished the enhancing effect of B6 on reprogramming ( Fig. 5g,h ). Collectively, these findings suggest that inhibition of AurkA kinase activity promotes GSK3β inactivation. Next, we sought to identify the kinase responsible for GSK3β phosphorylation following B6 treatment. Because Akt kinases are known to phosphorylate GSK3β, we asked whether Akt inhibitors interfered with the increase in phospho-GSK3β following treatment with B6. Indeed, treatment of 4F-infected MEFs with a small-molecule Akt inhibitor decreased the effect of B6 on GSK3β phosphorylation ( Fig. 6a ) and inhibited reprogramming ( Fig. 6b ). Moreover, phosphorylated Akt (Ser473) was increased in B6-treated cells ( Fig. 6c ), suggesting that the increased GSK3β phosphorylation seen following AurkA inhibition is mediated by Akt. We also tested the effects of 4F transduction and/or B6 treatment on the expression of several genes upstream of Akt, including Pdk1 , Src , Pten and p85α . However, we saw no significant changes in their mRNA levels when MEFs were transduced with 4F for 3 days and then treated with DMSO or B6 ( Fig. 6d ), indicating that B6 treatment does not alter transcription of Akt regulatory genes. 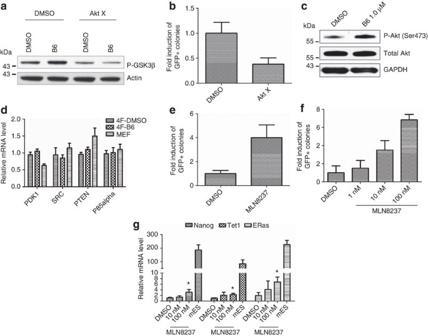Figure 6: B6-induced inactivation of GSK3β is mediated by Akt. (a) 4F-infected MEFs were treated with 1 μM each of Akt inhibitor (Akt X) and B6. GSK3β (Ser9) phosphorylation was diminished, most likely due to Akt inhibition. (b) Akt X inhibitor was added at a final concentration of 1 μM. Data are mean±s.d. of triplicate samples. (c) Inhibition of AurkA by B6 induces Akt phosphorylation on Ser473. MEFs were infected with 4F for 3 days and then treated with 1 μM B6 for two more days before collecting for western blotting analysis. GAPDH is glyceraldehyde 3-phosphate dehydrogenase. (d) B6 treatment does not alter expression of genes upstream of Akt. MEFs were transduced with 4F for 3 days and then treated with DMSO or 1 μM B6 for a further 2 days. Total RNA was collected and analysed pRT–qPCR for expression of the indicated genes, which have been reported to function upstream of Akt. Data are mean±s.d. of three independent wells. (e) AurkA inhibition by MLN8237 enhances reprogramming. 4F-infected MEFs were treated with 10 nM MLN8237 on day 3, and 10 days later GFP+ colonies were counted to determine reprogramming efficiency. MLN8237 enhanced iPSC generation similarly to the effect of 1 μM B6. Data are mean±s.d. from two experiments with triplicate samples. (f) MLN8237 dose-dependently enhances reprogramming. The number of Oct4-GFP+ colonies was significantly increased by MLN8237 treatment. Data are mean±s.d. of triplicate samples. (g) MLN8237 treatment induces mESC-specific gene expression in 4F-transduced MEFs. Cells were treated with DMSO or the indicated concentration of MLN8237 and collected on day 14 post-4F transduction for RT–qPCR analysis of Nanog, Tet1 and Eras. Data are mean±s.d. of three independent wells. *P<0.01 (Student'st-test). Figure 6: B6-induced inactivation of GSK3β is mediated by Akt. ( a ) 4F-infected MEFs were treated with 1 μM each of Akt inhibitor (Akt X) and B6. GSK3β (Ser9) phosphorylation was diminished, most likely due to Akt inhibition. ( b ) Akt X inhibitor was added at a final concentration of 1 μM. Data are mean±s.d. of triplicate samples. ( c ) Inhibition of AurkA by B6 induces Akt phosphorylation on Ser473. MEFs were infected with 4F for 3 days and then treated with 1 μM B6 for two more days before collecting for western blotting analysis. GAPDH is glyceraldehyde 3-phosphate dehydrogenase. ( d ) B6 treatment does not alter expression of genes upstream of Akt. MEFs were transduced with 4F for 3 days and then treated with DMSO or 1 μM B6 for a further 2 days. Total RNA was collected and analysed pRT–qPCR for expression of the indicated genes, which have been reported to function upstream of Akt. Data are mean±s.d. of three independent wells. ( e ) AurkA inhibition by MLN8237 enhances reprogramming. 4F-infected MEFs were treated with 10 nM MLN8237 on day 3, and 10 days later GFP+ colonies were counted to determine reprogramming efficiency. MLN8237 enhanced iPSC generation similarly to the effect of 1 μM B6. Data are mean±s.d. from two experiments with triplicate samples. ( f ) MLN8237 dose-dependently enhances reprogramming. The number of Oct4-GFP+ colonies was significantly increased by MLN8237 treatment. Data are mean±s.d. of triplicate samples. ( g ) MLN8237 treatment induces mESC-specific gene expression in 4F-transduced MEFs. Cells were treated with DMSO or the indicated concentration of MLN8237 and collected on day 14 post-4F transduction for RT–qPCR analysis of Nanog, Tet1 and Eras. Data are mean±s.d. of three independent wells. * P <0.01 (Student's t -test). Full size image To test the specificity of the effects of AurkA inhibition, we also determined whether MLN8237 enhanced iPSC generation. Treatment of MEFs with MLN8237 at a low concentration (10 nM) enhanced reprogramming approximately four fold and the effect was dose dependent ( Fig. 6e,f ). Gene expression analysis of MLN8237-treated samples also confirmed that the inhibitor increased expression of mESC-specific genes ( Fig. 6g ). As AurkA functions in the control of spindle formation and the cell cycle [33] , we determined whether treatment with AurkA inhibitors affected transition of 4F-infected MEFs through the cell cycle. We found that treatment of MEFs with various concentrations of B6 or MLN8237 had little effect on cell cycle progression ( Fig. 7a,b ), except that an increase in the number of cells in G2 was observed following treatment with high concentrations of MLN8237 (100 nM). This concentration of MLN8237 also significantly increased the number of GFP+ colonies and induced a mESC-specific gene expression profile ( Fig. 6f,g ). The size of the resulting colonies also resembled that of DMSO-treated cells, indicating that iPSC formation was not affected by MLN8237 at this dose, in contrast to fibroblast cells that undergo G2 arrest at this dose. 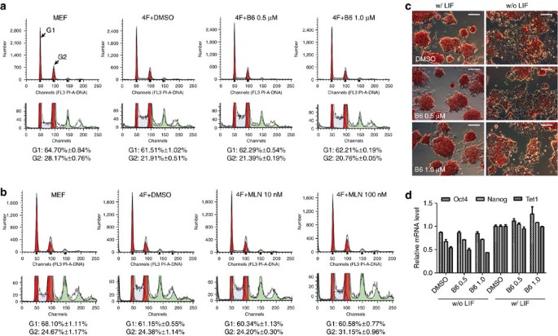Figure 7: Low level inhibition of AurkA does not affect MEFs cell cycle or mES differentiation. (a) 4F-infected MEFs were treated with different concentrations of B6 on day 3 post-infection. Cells were collected 48 h later, subjected to propidium iodide staining and analysed for DNA content by flow cytometry. (b) MLN8237 treatment at 10 nM did not alter the cell cycle of 4F-infected MEFs. The experimental procedure was as ina. (c) Aurora A kinase inhibitors do not inhibit mESC differentiation. Treatment with inhibitor B6 does not block changes in mESC morphology following LIF withdrawal. mESCs were cultured in LIF+ (w/LIF) or LIF−(w/oLIF) medium for 4 days and collected for AP staining. Differentiating cells become AP-negative and show a more scattered morphology. (d) Inhibitor B6 does not affect silencing of self-renewal genes following LIF withdrawal. The experimental procedure was as inc. Cells were collected for RNA extraction and RT–qPCR of the indicated mESC self-renewal genes. Data are mean±s.d. of triplicate samples. Figure 7: Low level inhibition of AurkA does not affect MEFs cell cycle or mES differentiation. ( a ) 4F-infected MEFs were treated with different concentrations of B6 on day 3 post-infection. Cells were collected 48 h later, subjected to propidium iodide staining and analysed for DNA content by flow cytometry. ( b ) MLN8237 treatment at 10 nM did not alter the cell cycle of 4F-infected MEFs. The experimental procedure was as in a . ( c ) Aurora A kinase inhibitors do not inhibit mESC differentiation. Treatment with inhibitor B6 does not block changes in mESC morphology following LIF withdrawal. mESCs were cultured in LIF+ (w/LIF) or LIF−(w/oLIF) medium for 4 days and collected for AP staining. Differentiating cells become AP-negative and show a more scattered morphology. ( d ) Inhibitor B6 does not affect silencing of self-renewal genes following LIF withdrawal. The experimental procedure was as in c . Cells were collected for RNA extraction and RT–qPCR of the indicated mESC self-renewal genes. Data are mean±s.d. of triplicate samples. Full size image AurkA is highly expressed in mESCs and iPSCs compared with MEFs [14] , suggesting that it functions to maintain mESC self-renewal or pluripotency. To determine whether inhibition of AurkA altered these properties, we treated mESCs with B6 at 0.5 or 1 μM and cultured the cells in the presence or absence of leukemia inhibitory factor (LIF) for 4 days. LIF withdrawal in both B6-treated and DMSO-treated control cells promoted mESC differentiation, as indicated by morphology and AP staining consistent with a loss of colonies ( Fig. 7c ). RT–qPCR confirmed that mESC differentiation was occurring, because self-renewal markers were downregulated in cells cultured in the absence of LIF ( Fig. 7d ). However, we did not see a significant effect of B6 treatment on either mESC self-renewal (in the presence of LIF) or differentiation (following LIF withdrawal), except a very small increase in Oct4 expression in mESCs. These results suggest that B6 treatment had little effect on iPSCs once they had reached the fully reprogrammed state. Since the first discovery that fibroblasts could be reprogrammed to iPSCs, great effort has been made to improve the extremely low efficiency of the process. A few small molecules have been shown to replace some 4F reprogramming factors in large-scale random screens [34] , whereas only a handful of compounds—most of which are chromatin-remodelling reagents—have been shown to enhance iPSC generation in 4F-infected cells. To date, TGF-β receptor inhibitors are the only kinase inhibitors known to directly enhance reprogramming [20] ; these compounds were shown to replace Sox2 and c-Myc by inducing Nanog expression [20] , an observation that led to the discovery that mesenchymal-to-epithelial transition is a key event during the early stages of reprogramming [21] , [22] . Thus, identifying kinases that function during reprogramming could not only provide targets to improve reprogramming efficiency but also provide insight into the molecular mechanisms of reprogramming. Here we report the results of an inhibitor screen designed to identify kinases important for reprogramming. We found that inhibition of P38, IP3K and AurkA significantly enhanced reprogramming efficiency, indicating that these kinases functioned as barriers to the process. Thus, modulation of the activities of these kinases, perhaps in combination with other currently available methods, could substantially increase reprogramming efficiency. Interestingly, we found that knockdown of p53 seemed to override the enhancing effects of these kinase inhibitors ( Supplementary Fig. S2g ). One potential explanation for this is that establishing an expedited ES-like cell cycle might be a fundamental requirement to reach the fully reprogrammed state. The kinase inhibitor treatments may have enhanced cell cycle progression among only a small percentage of the cells, which would not be easily detected in a mixed population. By contrast, knockdown of p53 would be expected to release the cell cycle arrest caused by oncogene overexpression, and thus the effects of the kinase inhibitors would likely not be observed. Our experiments have identified novel aspects of AurkA function, including inhibition of Akt-mediated phosphorylation and inactivation of GSK3β, which must be blocked to promote iPSC generation [35] . AurkA kinase has a well-characterized role in modulating centrosome function and spindle assembly [33] . Aberrant overexpression or reduced expression of AurkA also reportedly leads to tumour development [33] . We show that during reprogramming of MEFs to iPSCs, AurkA is highly induced even at an early stage (approximately day 5 post-4F transduction; Fig. 5b ), an event that correlated with the reduction of phospho-GSK3β in these cells ( Fig. 5e ). Modulating AurkA kinase activity could thus affect GSK3β activity and alter reprogramming efficiency. In addition, we saw that treatment with AurkA inhibitors increased AurkA protein levels. Recent studies indicate that AurkA may have kinase-independent functions, such as binding to and stabilizing N-MYC protein by blocking its ubiquitination [38] . N-MYC is also specifically expressed in mESCs or iPSCs, and recent work confirms that levels of endogenous N-MYC increase in reprogramming [14] . Interestingly, N-MYC degradation also requires sequential phosphorylation by cyclin B/Cdk1 and GSK3 [38] . Our screen also identified p38 and IP3K as barrier kinases. p38 reportedly regulates such diverse processes as the stress response, chromosome remodelling and the cell cycle [39] . Interestingly, p38 has been shown to have tumour suppressor function, and one of its regulatory targets is p53 (ref. 39 ). This observation could explain why p53 knockdown abolished the enhancing effect of a p38 inhibitor ( Supplementary Fig. S2g ). At the same time, p38 could also negatively regulate cell cycle progression [39] . Although we did not observe any effects of the inhibitors on growth of 4F-infected cells, we cannot rule out the possibility that a small percentage of cells gained a proliferative advantage following inhibition of p38, because very few cells reach a fully reprogrammed state. IP3K is the least studied of the proteins identified here as a barrier kinases. Gene expression profiles indicate that MEFs express low levels of IP3K but its expression is induced in partially reprogrammed iPSCs and iPS/mES cells [14] . IP3K functions primarily in calcium-dependent signal transduction [40] and its relationship to reprogramming requires further investigation. Our screen also identified kinases that function as potential enhancers of reprogramming. Specifically, we found that knockdown of the insulin-like growth factor (IGF) receptor Igf1r compromised reprogramming ( Fig. 3c ). Interestingly, IGF signalling reportedly activates the PI3K pathway, which can also activate Akt [41] . We have found that reprogramming is enhanced by knockdown of negative regulators of IGF signalling such as IGFBPs. These findings provide support for an important role for Akt function in iPSC generation. Although we found that the kinase inhibitors could enhance iPSC generation and that the reprogrammed cells reached a fully pluripotent state, it is not yet clear whether a specific cell population was affected by the inhibitors. Following expression of the four factors, a large number of unstable or partially reprogrammed cells never overcome the barrier to achieve a fully reprogrammed state. Do the kinase inhibitors accelerate the progression of unstable cells to the fully reprogrammed state or do they increase the starting pool of initiator cells for iPSC generation? Future work should identify the critical points at which the kinase inhibitors intervene in the reprogramming process. Collectively, our findings provide new insights into the molecular mechanisms by which somatic cells are reprogrammed into iPSCs, and we have identified new barrier genes that could serve as targets to design specific chemical inhibitors. Our study encourages further efforts to screen for small molecules that could prove useful in iPSC-based therapies. Cell culture and vectors Oct4-GFP MEFs were derived from mice carrying an IRES–EGFP fusion cassette downstream of the stop codon of pou5f1 (Jackson lab, Stock#008214) at E13.5. MEFs were cultured in DMEM (Invitrogen, 11995-065) with 10% FBS (Invitrogen) plus glutamine and NEAA. Only MEFs at passage 0–4 were used for reprogramming. pMX-Oct4, -Sox2, -Klf4 and -c-Myc were purchased from Addgene. Mouse AurkA was cloned into pMX. The human AurkA D274A mutant retroviral vector was purchased from Addgene. To generate retrovirus, Plat-E cells were seeded in 10-cm plates, and the next day cells were transfected with 9 μg of pMX-Oct4, -Sox2, -Klf4 and -c-Myc using Lipofectamine (Invitrogen, 18324-012) with PLUS reagent (Invitrogen, 11514-015). Viruses were collected 2 days later and combined. For reprogramming, MEFs were seeded in 12-well plates and the next day they were transduced with 4F virus using 4 μg ml −1 polybrene. One day later, the medium was replaced with fresh MEF medium, and 3 days later the medium was changed to mESC culture medium supplemented with LIF (Millipore, ESG1107). GFP+ colonies were picked on day 14 post-transduction, and expanded clones were cultured in DMEM with 15% FBS (Hyclone) plus LIF, thioglycerol, glutamine and NEAA. Irradiated CF1 MEFs served as feeder layers to culture mESC cells and derived iPSC clones. Kinase library screening A kinase library of 244 compounds was obtained from the chemical screening facility at the Sanford-Burnham Medical Research Institute. The library was purchased from Calbiochem (Library 1: 80 compounds, catalogue # 539744-1EA; Library 2: 80 compounds, catalogue # 539745-1EA; Library 3: 84 compounds, catalogue # 539746-1EA). All compounds are well-characterized protein kinase inhibitors. Compounds were diluted to 2 mM in 96-well plates. 4F-transduced cells were seeded into gelatin-coated plates (3,000 cells per well). Inhibitors were added at the indicated final concentrations every other day until day 13. Cells were then fixed with 4% paraformaldehyde for 20 min at room temperature (RT) and the number of Oct4-GFP+ colonies was directly counted under a microscope. Cells were then stained with Vector red AP substrate kit I (Vector laboratories, SK5100). siRNA transfection of MEFs siRNAs were purchased from Dharmacon and diluted in Opti-MEM (Invitrogen, 11058-021) to the desired final concentration. Lipofectamine 2000 (Invitrogen, 11668-019) was added to the mix at 2 μl per well in 12-well plates, which were incubated for 20 min at RT. For 12-well transfections, 80 μl of the siRNA/lipid mixture and 320 μl Opti-MEM was added to each well. Three hours later, 0.8 ml of the virus mixture (for iPSCs) or fresh medium was added to each well and the medium was changed to fresh MEF medium the next day. siRNAs were transfected twice during reprogramming (on days 0 and 5 post-4F transduction). Western blotting Total cell lysates were prepared by incubating cells in MPER buffer (Pierce, 78503) on ice for 20 min followed by centrifugation at 13,000 r.p.m. for 10 min. Equal volumes of lysate were resolved on 10% SDS–polyacrylamide gel electrophoresis gels, and the proteins were transferred to polyvinylidene difluoride membranes (Bio-Rad, 1620177) using the semi-dry system (Bio-Rad). Membranes were blocked with 5% milk in Tris-buffered Saline with Tween 20 (TBST). for at least 1 h at RT or overnight at 4 °C. Blots were then incubated with the following antibodies: anti-mNanog (R&D Systems, AF2729, 1:400), anti-h/mSSEA1 (R&D Systems, MAB2156, 1:400), anti-actin (Thermo Scientific, MS1295P0, 1:5,000), anti-AFP (Abcam, ab7751, 1:400), anti-β III tubulin (R&D Systems, MAB1368, 1:400), anti-α actin (Sigma, A7811, 1:400), anti-mAurkA (Bethyl Labs, A300-072A, 1:3,000), anti-hAurkA (Bethyl Labs, A300-071A, 1:1,000), anti-total-GSK3β (Cell Signaling Technology, 9315S, 1:1,000), anti-phospho-GSK3β (Ser9) (Cell Signaling Technology, 9323S, 1:1,000), anti-total Akt (Cell Signaling Technology, 9272S, 1:1,000) and anti-phospho-Akt (Ser473) (Cell Signaling Technology, 9271S, 1:1,000). Quantitative reverse transcription–PCR Total RNA was extracted using Trizol (Invitrogen). After extraction, 1 μg total RNA was used for reverse transcription using Superscript II (Invitrogen). Quantitative PCR was performed using a Roche LightCycler480 II (Roche) and the SYBR green mixture from Abgene (Ab-4166). Gene primers are listed in Supplementary Table S2 . Immunostaining Cells were washed twice with PBS and fixed with 4% paraformaldehyde at RT for 20 min. Fixed cells were permeabilized with 0.1% Triton X-100 for 5 min. Cells were then blocked in 5% BSA/PBS containing 0.1% Triton X-100 for 1 h at RT. Primary antibodies were diluted between 1:100 and 1:400 in 2.5% BSA/PBS containing 0.1% Triton X-100, according to the manufacturer's suggestion. Cells were stained with primary antibody for 1 h and then washed three times with PBS. Secondary antibodies were diluted 1:400 and incubated with cells for 45 min at RT. EB formation and differentiation assay iPSCs were trypsinized into a single-cell suspension and the hanging drop method was used to generate EBs. Each drop consisted of 4,000 iPSCs in 20 μl EB differentiation medium. EBs were cultured in hanging drops for 3 days before being reseeded onto gelatin-coated plates. After reseeding, cells were further cultured until day 14, when beating areas could be identified. Teratoma formation and chimera generation iPSCs were trypsinized and resuspended at 1×10 7 cells per ml. Athymic nude mice were anaesthetized with Avertin, and ~150 μl of the cell suspension was injected into each mouse. Mice were examined for tumours every week for 3–4 weeks. Tumours were collected and fixed in zinc formalin solution for 24 h at RT before being paraffin embedded and stained with hematoxylin and eosin. To test the capacity of derived iPSC clones to contribute to chimeras, iPSCs were injected into C57BL/6J-Tyr (C-2J)/J (albino) blastocysts. Generally, each blastocyst received 12–18 iPSCs. Imprinting control region (ICR)-recipient females were used for embryo transfer. Donor iPSCs confer agouti or black coat colour. All animal work and use of animals complied with institutional regulations. mRNA microarray analysis Total RNA was extracted from derived iPSCs using Trizol. mRNA microarray analysis was carried out by the microarray facility at the Sanford-Burnham Medical Research Institute. ArrayExpress accession: E-MTAB-1188 . A scatter plot was used to compare the genome-wide mRNA expression profiles of iPSCs, MEFs and mESCs. Cell proliferation assay MEFs were seeded at 3,000 cells per well in 96-well plates and transduced with 4F virus for 3 days. Cells were treated with inhibitors at 0.5 μM. Proliferation was measured every other day by incubating cells with mESC medium containing CellTiter 96 Aqueous One solution (Promega, G3580) for 1 h at 37 °C. Absorbance at 490 nm was measured using a plate reader, and relative proliferation curves were constructed using the absorbance signal from day 3 post-4F transduction as a reference. Cell cycle analysis Control or 4F-infected MEFs were treated with inhibitors for 2 days and then collected, trypsinized and fixed in 75% ethanol overnight. Cells were centrifuged at 1,000 r.p.m. for 5 min, washed once with PBS and incubated with propidium iodide staining solution for at least 30 min at RT before flow cytometric analysis. Approximately 20,000 events were collected per sample and cell cycle data were modelled using ModFit software. Accession codes: The microarray data have been deposited in ArrayExpress under the accession code E-MTAB-1188 . How to cite this article: Li, Z. & Rana, T.M. A kinase inhibitor screen identifies small-molecule enhancers of reprogramming and iPS cell generation. Nat. Commun. 3:1085 doi: 10.1038/ncomms2059 (2012).